Evidence for fungal and chemodenitrification based N2O flux from nitrogen impacted coastal sediments Although increasing atmospheric nitrous oxide (N 2 O) has been linked to nitrogen loading, predicting emissions remains difficult, in part due to challenges in disentangling diverse N 2 O production pathways. As coastal ecosystems are especially impacted by elevated nitrogen, we investigated controls on N 2 O production mechanisms in intertidal sediments using novel isotopic approaches and microsensors in flow-through incubations. Here we show that during incubations with elevated nitrate, increased N 2 O fluxes are not mediated by direct bacterial activity, but instead are largely catalysed by fungal denitrification and/or abiotic reactions (e.g., chemodenitrification). Results of these incubations shed new light on nitrogen cycling complexity and possible factors underlying variability of N 2 O fluxes, driven in part by fungal respiration and/or iron redox cycling. As both processes exhibit N 2 O yields typically far greater than direct bacterial production, these results emphasize their possibly substantial, yet widely overlooked, role in N 2 O fluxes, especially in redox-dynamic sediments of coastal ecosystems. Nitrogen (N) loading from anthropogenic activities profoundly impacts ecosystems worldwide, with loading to coastal zones among the largest challenges facing humanity, as nearly half the global population lives within 100 km of the coast. Coastal sediments are known hotspots of biogeochemical transformations and recognized as effective agents for removing excess nitrogen [1] , [2] . However, biological removal of reactive nitrogen may also occur at the expense of increased production of nitrous oxide (N 2 O), a potent climatically active trace gas. Despite being the largest ozone depleting substance currently emitted to the atmosphere [3] , N 2 O remains unregulated by the international community and large uncertainties exist concerning N 2 O budgets (>100%), particularly for heterogeneous environments such as coasts [4] , [5] . Redox-dynamic estuarine and coastal sediments routinely experience high N loading and low dissolved oxygen (O 2 ), conditions that are strongly linked to elevated N 2 O and underlie their estimated 10% contribution to the global N 2 O flux [4] , [6] , [7] , [8] , [9] . Thus, understanding their role in both nitrogen removal and N 2 O production is important for improving predictions of long-term impacts of human activity across globally relevant scales. Many studies have focused on the relative contribution of bacterial denitrification (bDNF) or nitrification (oxidation of ammonia (NH 3 ) to nitrite (NO 2 − ) or ‘AMO’), as controlling processes underlying N 2 O emissions ( Fig. 1 ). While yields of N 2 O from both AMO and bDNF are low (<1% in terms of total moles of N converted), their magnitude and ubiquity across ecosystems translates into major atmospheric fluxes. Increasingly, however, the potential for other N 2 O production processes has become apparent, including production of N 2 O by fungi and/or abiotic reactions coupled to redox cycling of metals such as iron [10] , [11] , [12] . In particular, the organic-rich and redox-dynamic regimes of estuarine and coastal sediments may promote both fungal activity and rapid redox cycling of iron. To examine controls and mechanisms of N 2 O production in coastal sediments ( Fig. 1 ), we incubated natural sediment cores under flow-through conditions, manipulating both dissolved O 2 and nitrate in the overlying water (using conditions typifying anthropogenically impacted ecosystems), while monitoring both porewater N 2 O profiles and stable isotopic fluxes of ammonium, nitrate, nitrite and N 2 O. Given the complexity of processes involved, we also leveraged the use of a less-traditional isotope system ( 17 O, described below) to provide even broader perspective for disentangling operative N 2 O cycling mechanisms. 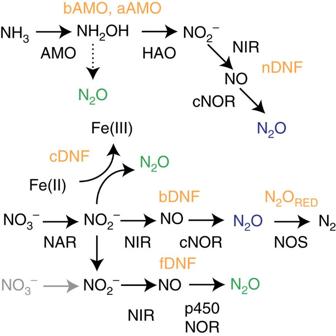Figure 1: Schematic representation of N2O production pathways considered in this study. N2O can form during decomposition/reaction of intermediate hydroxylamine (NH2OH) produced during ammonia oxidation by bacteria (bAMO) or archaea (aAMO). Some of these nitrifying organisms may also produce N2O during reduction of product nitrite (NO2−), known as nitrifier-denitrification (nDNF). N2O may also be produced during reduction of nitrate and/or nitrite by denitrification catalysed by bacteria (bDNF), fungi (fDNF) and/or by chemical reaction with Fe(II) or ‘chemodenitrification’ (cDNF). Finally, N2O can also be reductively consumed by denitrifying bacteria (N2ORED). N2O produced having low or negative site preference values (−10 to 0‰) are indicated in blue, while those have high site preference values (>15‰) are indicated in green. Enzymes are indicated as ammonia monooxygenase (AMO), hydroxylamine oxidoreductase in bacterial nitrification (HAO), nitrate reductase (NAR), nitrite reductase (NIR), bacterial nitric oxide reductase (cNOR), nitrous oxide reductase (NOS) and fungal nitric oxide reductase (p450NOR). The detailed biochemical pathway of nitrite production by archaeal ammonia oxidation remains unclear. Figure 1: Schematic representation of N 2 O production pathways considered in this study. N 2 O can form during decomposition/reaction of intermediate hydroxylamine (NH 2 OH) produced during ammonia oxidation by bacteria (bAMO) or archaea (aAMO). Some of these nitrifying organisms may also produce N 2 O during reduction of product nitrite (NO 2 − ), known as nitrifier-denitrification (nDNF). N 2 O may also be produced during reduction of nitrate and/or nitrite by denitrification catalysed by bacteria (bDNF), fungi (fDNF) and/or by chemical reaction with Fe(II) or ‘chemodenitrification’ (cDNF). Finally, N 2 O can also be reductively consumed by denitrifying bacteria (N 2 O RED ). N 2 O produced having low or negative site preference values (−10 to 0‰) are indicated in blue, while those have high site preference values (>15‰) are indicated in green. Enzymes are indicated as ammonia monooxygenase (AMO), hydroxylamine oxidoreductase in bacterial nitrification (HAO), nitrate reductase (NAR), nitrite reductase (NIR), bacterial nitric oxide reductase (cNOR), nitrous oxide reductase (NOS) and fungal nitric oxide reductase (p450NOR). The detailed biochemical pathway of nitrite production by archaeal ammonia oxidation remains unclear. Full size image The steady-state emission flux of N 2 O ( F N2O ) is governed by six possible production fluxes (F) ( Fig. 1 ; bacterial denitrification (bDNF), fungal denitrification (fDNF), chemodenitrification (cDNF; specifically the abiotic reduction of NO 2 − to N 2 O by Fe(II)), ammonia oxidation by bacteria (bAMO) or archaea (aAMO) and nitrifier-denitrification (nDNF)), as well as respiratory consumption by denitrifying bacteria (N 2 O RED ) such that: Stable isotopes of N 2 O have been widely used for studying its production and consumption, including both oxygen ( 18 O/ 16 O) and bulk nitrogen ( 15 N/ 14 N) (δ=((( R sample / R standard )−1) × 1,000) and R = 15 N/ 14 N or 18 O/ 16 O) [13] , [14] , [15] , [16] , [17] , [18] , [19] . In addition, the unique intra-molecular distribution of 15 N within N 2 O molecules has emerged as a powerful tool for constraining N 2 O cycling, as differences in 15 N content between the central ‘α’ and outer ‘β’ atoms of the N 2 O molecule (‘site preference’ or SP N2O , where SP N2O =δ 15 N α −δ 15 N β ) have been shown to reflect formation pathways [13] , [14] , [16] , [18] . Numerous studies have measured the steady-state δ 15 N offset between precursor molecules (NO 3 − , NO 2 − and NH 4 + ) and N 2 O (‘Δδ 15 N’=δ 15 N source −δ 15 N N2Obulk ), as well as SP N2O values towards characterizing signature compositions for the processes in equation 1. Some compositional overlap notwithstanding, the isotopic separation of many of these endmembers has been used to distinguish their relative contribution to N 2 O production, especially nitrification and denitrification [14] , [19] , [20] . Notably, the respiratory reduction of N 2 O by denitrifying bacteria can increase the δ 15 N bulk of the remaining N 2 O (decreasing Δδ 15 N values), as well as SP N2O values (with a distinctive relationship between isotope effects imparted on the δ 15 N of the bulk N 2 O and its site preference, 15 ɛ bulk and SP ɛ, respectively [21] , [22] ) modifying mixing relationships. Nevertheless, measured values of Δδ 15 N and SP N2O are quantitative integrators of the proportion of each process (which may then be modified by N 2 O reduction; see Methods), serving as independently responsive tracers for constraining production mechanisms. To further interrogate N 2 O dynamics, we also used a natural atmospherically derived NO 3 − having an unusual triple oxygen isotopic composition (containing excess 17 O) that provides novel ‘isotope space’ for further resolving co-occurring processes. By comparing levels of 17 O-excess within discrete N pools (see Methods), we are able to independently quantify the proportion of N 2 O deriving from NO 3 − (or NO 2 − ) and thereby, in concert with the more conventional isotopic measurements (Δδ 15 N, SP), uniquely explain variations in N 2 O producing pathways. Below we summarize our results, combining microprofile perspectives with the use of these mass and isotopic fluxes to constrain N 2 O production mechanisms in coastal sediments of the Wadden Sea under a variety of incubation conditions ( Supplementary Fig. 1 ). Specifically, we find that the isotopic composition of increased N 2 O fluxes resulting from elevated nitrate loading in our incubations requires substantial contribution by processes not regularly considered in coastal ecosystems, namely fungal and/or chemodenitrification. We suggest that variations in the contribution of these processes to N 2 O fluxes from coastal and other ecosystems may help to explain the notorious variability that is frequently encountered in studies of N 2 O dynamics. Microsensor and mass flux perspectives on N 2 O Microsensor profiles revealed shallow O 2 penetration ( ∼ 2–3 mm) typical of high-respiration rates occurring in organic-rich sediments, with occasional subsurface peaks in O 2 reflecting bioturbation/bioirrigation ( Fig. 2a ). N 2 O profiles revealed striking vertical and lateral heterogeneity in location, magnitude and distribution of N 2 O, reflecting the complexity of N 2 O dynamics ( Fig. 2b–f ). Elevated N 2 O was often observed near the sediment–water interface, suggesting oxidative production by AMO. However, zones of extremely elevated N 2 O (>3 μM, not shown) were also observed much deeper, highlighting its spatial heterogeneity. In some cases, subsurface N 2 O appeared connected with the overlying water, co-occurring near subsurface O 2 peaks and reflecting oxidative N 2 O production despite reducing surroundings. In others, elevated N 2 O coincided with anoxic conditions, suggesting N 2 O production by reductive pathways ( Fig. 2b ). Several cores had active burrows extending into the sediment, likely contributing to this heterogeneity. In part, these observations extend the view of N 2 O dynamics to slightly deeper sediment layers, in contrast to previous observations mostly focusing on dynamics in the upper 1 cm (refs 23 , 24 ). This remarkable heterogeneity, often even laterally within a single core, hinders straightforward N 2 O flux calculations, yet emphasizes the utility of the whole core incubation stable isotope approach, which integrates this natural heterogeneity and provides a complementary and mechanistic perspective on underlying N 2 O dynamics. 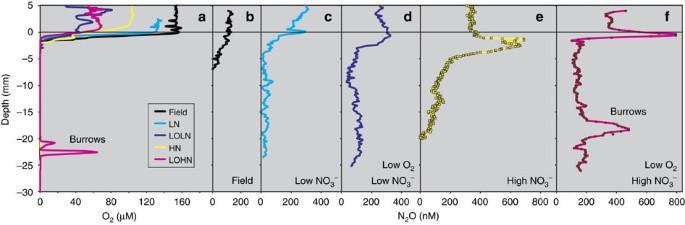Figure 2: Example microsensor profiles of O2and N2O from sediment core incubations from the Mischwatt site illustrating typical heterogeneity observed. Rapid consumption of O2in the upper 2–3 mm (a) reflects the high organic matter content and respiration rates of these sediments. Depth profiles of N2O are shown inbthroughf. ‘Field’ profile (b) reflects conditions immediately upon core collection. Profiles from experiment cores reflect porewater conditions after∼7–8 days of incubation under low NO3−(c), low O2and low NO3−(d), high NO3−(e) and low O2and high NO3−(f). The complexity in the structure of the N2O profiles—including subsurface zones of production likely influenced by bioirrigation—complicate their use in conventional flux estimation by porewater models. Figure 2: Example microsensor profiles of O 2 and N 2 O from sediment core incubations from the Mischwatt site illustrating typical heterogeneity observed. Rapid consumption of O 2 in the upper 2–3 mm ( a ) reflects the high organic matter content and respiration rates of these sediments. Depth profiles of N 2 O are shown in b through f . ‘Field’ profile ( b ) reflects conditions immediately upon core collection. Profiles from experiment cores reflect porewater conditions after ∼ 7–8 days of incubation under low NO 3 − ( c ), low O 2 and low NO 3 − ( d ), high NO 3 − ( e ) and low O 2 and high NO 3 − ( f ). The complexity in the structure of the N 2 O profiles—including subsurface zones of production likely influenced by bioirrigation—complicate their use in conventional flux estimation by porewater models. Full size image In contrast to the oxidative N 2 O production captured by the micro-profiles at the sediment–water interface, mass fluxes suggest an important role for reductive N 2 O production. Nitrate levels in the overlying water were closely related to N 2 O flux from the sediment, with net efflux of N 2 O from the sediment in all cases ranging from 1.4 up to 84.2 μmoles m −2 d −1 ( Table 1 ; Supplementary Fig. 1 ; Supplementary Table 2 ). While fluxes of N 2 O under low nitrate conditions averaged 17.8 μmoles m −2 d −1 ( Table 1 ), decreasing dissolved O 2 saturation to ∼ 30% reduced N 2 O fluxes (5.9 μmoles m −2 d −1 ). In contrast, addition of NO 3 − to the overlying water significantly increased N 2 O (as well as NO 2 − ) fluxes ( Table 1 ) to the water column, consistent with other studies linking elevated coastal NO 3 − loading with efflux of N 2 O to the atmosphere [6] , [8] , [25] . Corresponding NO 3 − consumption also increased significantly, reflecting diffusion-limitation of organic matter respiration ( Table 1 ; Supplementary Fig. 1 ; Supplementary Table1 ). Table 1 Steady state mass fluxes of measured nitrogen species. Full size table Multi-isotope analysis of underlying N 2 O cycling processes The stable isotopic composition of N 2 O and other nitrogen pools ( Table 2 ; Supplementary Table 2 ) provides additional insight into specific biogeochemical mechanisms regulating sedimentary N 2 O fluxes. Average SP N2O for low-nitrate (LN) and low-O 2 /low-nitrate (LOLN) experiments were not significantly different (7.2±3.4 and 6.2±3.2‰, respectively) and, together with small differences between effluent NO 3 − and N 2 O δ 15 N (Δδ 15 N) indicate that N 2 O fluxes were largely linked to bacterial denitrification (having low SP N2O ) that was limited by diffusive supply of NO 3 − (yielding low Δδ 15 N) ( Fig. 3 ), a common characteristic of organic-rich sediments [26] . Notably, SP N2O values were higher than values expected from bDNF alone, however, reflecting contribution by additional N 2 O cycling processes. Table 2 Steady state isotopic composition of measured nitrogen species. 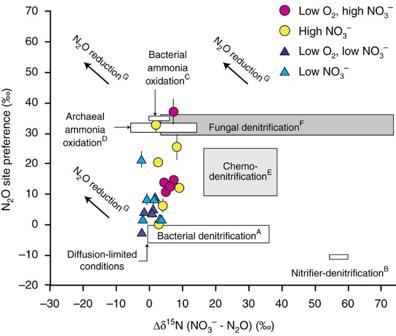Figure 3: Multiple isotope plot of N2O illustrating predicted compositional fields of various processes as well as steady-state composition of N2O fluxes from incubations. For illustrating representative compositional fields of N2O production processes (boxes), ranges are taken from literature reports of the offset between precursor molecule and predicted N2O (Δδ15N, or the difference in δ15N between NH4+and N2O for bacterial and archaeal ammonia oxidation, between NO2−and N2O for chemodenitrification or between NO3−and N2O for denitrification). References (in parentheses) include for (A) bacterial denitrification20,83,84, (B) nitrifier-denitrification59, (C) bacterial ammonia oxidation20,59,84,85, (D) archaeal ammonia oxidation56,57,58, (E) chemodenitrification47,48,49, (F) fungal denitrification37,42,43,44and (G) bacterial N2O reduction21,22,86, which has been shown to result in a coupled increase in δ15N and SP of the remaining N2O pool (indicated by arrows). Experimentalx-axis data are δ15NNO3–δ15NN2O. Error bars in they-direction are 1 s.d., while in thex-direction error is smaller than the symbols. Note that for mass balance calculations the actual measured steady-state isotope values of precursor molecules (for example, NH4+or NO3−) were used as appropriate for constraining endmember values of each process. In general, addition of∼100 μM NO3−to the overlying water increased N2O fluxes with an accompanying increase in N2O site preference, while not decreasing the Δδ15N (as would be expected from N2O reduction, arrows), implicating an increased production of N2O from a process deriving from NO3−(or NO2−) yet also one yielding an elevated site preference such as chemodenitrification and/or fungal denitrification. Full size table Figure 3: Multiple isotope plot of N 2 O illustrating predicted compositional fields of various processes as well as steady-state composition of N 2 O fluxes from incubations. For illustrating representative compositional fields of N 2 O production processes (boxes), ranges are taken from literature reports of the offset between precursor molecule and predicted N 2 O (Δδ 15 N, or the difference in δ 15 N between NH 4 + and N 2 O for bacterial and archaeal ammonia oxidation, between NO 2 − and N 2 O for chemodenitrification or between NO 3 − and N 2 O for denitrification). References (in parentheses) include for (A) bacterial denitrification [20] , [83] , [84] , (B) nitrifier-denitrification [59] , (C) bacterial ammonia oxidation [20] , [59] , [84] , [85] , (D) archaeal ammonia oxidation [56] , [57] , [58] , (E) chemodenitrification [47] , [48] , [49] , (F) fungal denitrification [37] , [42] , [43] , [44] and (G) bacterial N 2 O reduction [21] , [22] , [86] , which has been shown to result in a coupled increase in δ 15 N and SP of the remaining N 2 O pool (indicated by arrows). Experimental x -axis data are δ 15 N NO3 –δ 15 N N2O . Error bars in the y -direction are 1 s.d., while in the x -direction error is smaller than the symbols. Note that for mass balance calculations the actual measured steady-state isotope values of precursor molecules (for example, NH 4 + or NO 3 − ) were used as appropriate for constraining endmember values of each process. In general, addition of ∼ 100 μM NO 3 − to the overlying water increased N 2 O fluxes with an accompanying increase in N 2 O site preference, while not decreasing the Δδ 15 N (as would be expected from N 2 O reduction, arrows), implicating an increased production of N 2 O from a process deriving from NO 3 − (or NO 2 − ) yet also one yielding an elevated site preference such as chemodenitrification and/or fungal denitrification. Full size image In contrast, the increased N 2 O fluxes under elevated NO 3 − exhibited higher SP N2O relative to low nitrate experiments, averaging 16.2±5.0 and 12.9±2.5‰ for the high-nitrate (HN) and low-O 2 /high nitrate (LOHN), respectively ( Fig. 3 , Table 2 ), and indicating a shift in N 2 O dynamics. This increase in SP N2O , however, was not accompanied by an increase in δ 15 N of the N 2 O pool (no apparent decrease in Δδ 15 N), as would be expected by increased N 2 O reduction [21] , [27] . This observation implicates the stimulation of processes that produce N 2 O with high SP N2O —namely, b/aAMO, fDNF and/or cDNF. Below, we use the triple oxygen isotopes of co-existing NO 3 − , NO 2 − and N 2 O to further examine these candidate processes responding to elevated NO 3 − loading. Triple oxygen isotopes as a tool for constraining nitrogen cycling Our multi-pool Δ 17 O measurements enable disentangling of processes that are otherwise overlapping (in SP N2O values, for example), providing a complementary perspective to the N isotope analyses. First, these analyses revealed that nitrification played a relatively small role in NO 3 − production. As noted, amended nitrate had a high Δ 17 O NO3 value (+18.5‰), which when combined with pre-existing nitrate in the supply seawater (Δ 17 O NO3 =0‰) yielded a Δ 17 O NO3 of ∼ +15.3‰ ( Table 2 ). As changes to this Δ 17 O NO3 value occur only by production of new nitrate during nitrification [28] , [29] , the small differences in Δ 17 O NO3 between the inflow and effluent (at most 0.8‰; Table 2 ), reflect small relative contribution of newly produced NO 3 − by nitrification. Comparatively, Δ 17 O N2O values averaged +6.5 and +5.4‰ for high nitrate (HN) and low O 2 /high nitrate (LOHN), respectively. These are lower than the corresponding Δ 17 O NO3 ( Table 2 ), yet unequivocally reflect transfer of NO 3 − derived O atoms into the N 2 O flux. Whether the lower Δ 17 O N2O (relative to Δ 17 O NO3 ) stems from production of N 2 O by processes having a precursor other than NO 3 − (for example, bAMO/aAMO) or from the equilibration of intermediate NO 2 − with water (also causing Δ 17 O to approach 0‰) cannot be ascertained by comparing Δ 17 O NO3 and Δ 17 O N2O (equation 2). However, Δ 17 O NO2 values were also typically lower than steady-state Δ 17 O NO3 , averaging +8.5 and +9.2‰, respectively ( Table 2 ). While non-zero Δ 17 O NO2 values reflect reduction of NO 3 − to NO 2 − (since Δ 17 O is conserved), Δ 17 O NO2 values lower than steady-state Δ 17 O NO3 values must reflect NO 2 − production by ammonia oxidation (bAMO or aAMO) and/or partial equilibration of NO 2 − with water. Regardless, comparison of steady-state Δ 17 O N2O with Δ 17 O NO2 (equation 5) indicates an average of 70–80% of the N 2 O derived from a NO 2 − precursor under high NO 3 − incubations and thus indicates that the increased production occurred via reductive pathways ( Fig. 4 ) and not by a/bAMO. Together with the elevated SP N2O and only small changes in Δδ 15 N, this suggests fungal and/or chemodenitrification as possible contributors ( Fig. 4 ). Both fDNF and cDNF are dependent on supply of NO 2 − and typically exhibit yields far greater than bacterial N 2 O production (that is, the relative amount of N 2 O emitted per mole of NO 3 − or NO 2 − reduced or NH 3 oxidized). Thus, only small levels of these processes would be required to contribute relatively large amounts of N 2 O—setting the stage for a potentially important role for these biogeochemical processes in regulating N 2 O fluxes wherever they occur. 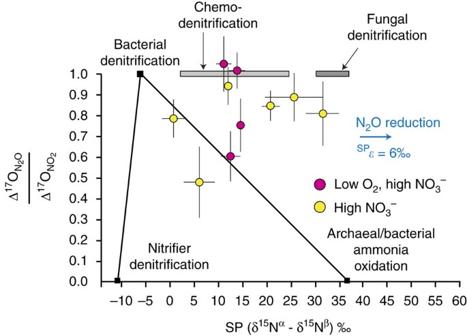Figure 4: Comparison of steady state triple oxygen isotope composition of N2O and NO2−with SPN2Ofor experiments amended with NO3−. Endmember composition for they-axis was based on the assumption that bacterial, fungal and chemodenitrification are utilizing the steady-state NO2−pool as a substrate (where Δ17ONO2=steady-state value), while nitrifier-denitrification uses only NO2−derived directly from NH4+oxidation (Δ17ONO2=0‰). Increases in SPN2Ovalues may be caused by N2O reduction (Ostromet al.21; Jinuntuya-Nortmanet al.86), however, this mass dependent process will only impact SPN2Oand not alter Δ17O values (horizontal arrow). Error bars represent±1σfor SPN2Oand propagated error for Δ17ON2O/Δ17ONO2. Data demonstrate that associated increases in SPN2Oupon elevated NO3−is not associated with ammonia oxidation, but instead is linked to increased contribution of fungal and/or chemodenitrification. Figure 4: Comparison of steady state triple oxygen isotope composition of N 2 O and NO 2 − with SP N2O for experiments amended with NO 3 − . Endmember composition for the y -axis was based on the assumption that bacterial, fungal and chemodenitrification are utilizing the steady-state NO 2 − pool as a substrate (where Δ 17 O NO2 =steady-state value), while nitrifier-denitrification uses only NO 2 − derived directly from NH 4 + oxidation (Δ 17 O NO2 =0‰). Increases in SP N2O values may be caused by N 2 O reduction (Ostrom et al . [21] ; Jinuntuya-Nortman et al . [86] ), however, this mass dependent process will only impact SP N2O and not alter Δ 17 O values (horizontal arrow). Error bars represent±1 σ for SP N2O and propagated error for Δ 17 O N2O /Δ 17 O NO2 . Data demonstrate that associated increases in SP N2O upon elevated NO 3 − is not associated with ammonia oxidation, but instead is linked to increased contribution of fungal and/or chemodenitrification. Full size image Diversity and abundance of fungi in oxygen-depleted coastal sediments is generally thought to represent a small fraction of their soil-hosted counterparts [30] , [31] , [32] . Nevertheless, their ecological role remains unclear—with recent studies challenging the perspective that fungi are only ecologically significant under aerobic conditions [31] , [32] , [33] . Adapted for organic-rich environments often depleted in O 2 , many fungi have a range of cellular adaptations to life under suboxic conditions [32] , [34] , [35] , [36] , including the ability to couple denitrification [37] directly to mitochondrial respiration [38] —a metabolic capacity that has been documented in a variety of environments including coastal sediments [34] , [39] . Given this respiratory flexibility, fDNF is poised to be especially important under hypoxic conditions and wetland environments, where access to O 2 in overlying water is juxtaposed with anoxic, carbon-rich conditions [40] . The most characteristic feature of the fungal-denitrifying system is a P450 cytochrome operating as a nitric oxide reductase (P450nor) [41] giving rise to the characteristically high SP of ∼ 35–37‰ (refs 42 , 43 ), the biochemical nature of which was recently interrogated in the purified enzyme [44] . Although assessment of fungal metabolic activity was beyond our scope, sequencing of the fungal ITS region revealed the presence of fungi across all incubations and study sites ( Supplementary Fig. 3 ), indicating diverse sequences including members of several divisions, some of which include N 2 O producing isolates [37] . While their presence does not confirm specific physiological activity involved in nitrogen transformations, taken together our results point to an unexplored role of fungi in coastal sedimentary N cycling. In particular, as fungi lack N 2 O reductase [38] , yields from fDNF are also typically 1–2 orders of magnitude greater than for bDNF (generally <0.1%) and N 2 O production appears to be physiologically widespread among fungi [37] . Indeed the importance of fungi in contributing to N 2 O production is well-recognized across a range of terrestrial ecosystems [45] . While their overall role in the reductive elimination of reactive N may be small relative to that of bacterial denitrification, these high yields mean that even small levels of fDNF could have disproportionately large impacts on N 2 O release, serving as an important, yet under-recognized source to the atmosphere. Although biological N 2 O production has received much attention, abiotic production of N 2 O is also widely documented, typically via reactions involving intermediates such as NH 2 OH and NO 2 − —though its environmental role remains unclear (Zhu-Barker et al . [11] , and references therein). Specifically, reduced iron (Fe(II)), especially mineral or surface-bound Fe(II), is an effective catalyst of NO 2 − reduction under a range of conditions [46] , and the presence of mineral surfaces and elevated levels of Fe(II) has also been shown to increase N 2 O yield [47] , [48] . Although data are limited, SP N2O from chemodenitrification is generally >10‰ and recent evidence suggests that elevated reaction rates, promoted by high levels of Fe(II), may also increase SP N2O (up to 26‰) ( [47] , [48] , [49] , [50] , [51] ). The production of reactive Fe(II) as the result of direct or indirect microbial activity is a ubiquitous feature of marine sediments. Our sites contained between 67 and 1344 μM HCl-extractable Fe(II) g −1 wet sediment ( Supplementary Fig. 4 ). However, prediction of reaction kinetics between Fe(II) and NO 2 − in these porewater environments is complex, particularly given the range of binding environments of Fe(II), which largely controls its reactivity [52] , [53] . Nonetheless, the positive flux of NO 2 − together with the porewater Fe(II) levels suggests that cDNF may also have contributed to N 2 O production. Interestingly, however, despite its lower Fe(II), the sandy site (SD) exhibited similar overall N 2 O isotope dynamics to the other two more Fe-rich sites ( Table 2 ), suggesting that perhaps the increased response of N 2 O production to NO 3 − loading was perhaps not as tightly linked to Fe(II) content. On the basis of the isotope systematics described, we use an isotope mass balance (based on equations 1, 2, 5 and 6 and defined endmember compositions ( Supplementary Table 3 )) to estimate relative contribution of operative N 2 O producing mechanisms (see Methods). While fDNF and cDNF are not mutually exclusive, we consider them separately to more robustly evaluate their potential contribution. Previous studies appear to demonstrate a strong relative dominance of ammonia oxidizing bacterial abundance compared to archaea in organic-rich coastal sediments [54] , [55] . An assumed numerical dominance of bacterial ammonia oxidizers notwithstanding, pure culture studies of archaeal ammonia oxidizers typically produce N 2 O reflecting a isotopic compositional mixture of both the AMO and nDNF pathways [56] , [57] , [58] , as has been more directly characterized in bacterial ammonia oxidizers [59] . Ongoing studies of N 2 O production mechanisms in ammonia oxidizing archaea will undoubtedly provide more insight on their unique biochemical nature. Differences in biochemistry aside, however, given the apparent similarity in isotopic composition of N 2 O deriving from bAMO and aAMO (especially a high SP N2O value, Figs 3 and 4 ), here we opt to combine bacterial and archaeal AMO for consideration in our mass balance analysis—setting endmember values to those previously determined for bAMO, as these have been studied in far more detail [59] . Thus, for elevated nitrate experiments (in which we can leverage the use of the positive Δ 17 O), we consider N 2 O production by bDNF, nDNF and AMO (bAMO+aAMO) together with either fDNF or cDNF ( Supplementary Table 4 ), while also examining the relative influence of N 2 O reduction on the calculated steady-state contributions of each process (see Methods). Error was estimated using a Monte Carlo approach in R with 10,000 simulations ( Supplementary Table 4 ; see Supplementary Information for a more detailed sensitivity analysis of endmember composition). Under elevated nitrate, mass balance indicates N 2 O production predominantly driven by varying contribution of bacterial and fungal denitrification ( Fig. 5 ; Supplementary Table 4 ). For the base case ( Supplementary Table 3 ), fungal denitrification contributed on average 36% of the N 2 O flux (up to 70% in one core). 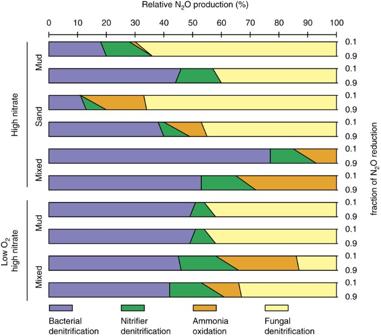Figure 5: Relative contribution of N2O produced by four cycling processes as calculated by N2O isotope mass balance. Each bar reflects steady-state calculations using measurements from a single core incubation (two cores were incubated per site per treatment and are shown separately), considering bacterial denitrification, ammonia oxidation, nitrifier denitrification and fungal denitrification. For illustration of the relative influence that N2O reduction (and its associated isotope fractionation) plays in the mass balance estimates, scenarios of both low (10%, upper) and high (90%, lower) relative N2O consumption are considered for each core (right side axis). Contribution by processes where mass balance estimates yielded small negative values (Supplementary Table 4) were considered equal to zero for this figure, with other values weighted accordingly to sum to 100%. The reader is also referred toSupplementary Table 4for associated error in mass balance estimates calculated by Monte Carlo simulation, as well asSupplementary Tables 5 and 6for sensitivity analyses of alternative endmember compositions. In evaluating the sensitivity of these estimates to endmember composition, this average value increased to 41 or 56% (if using a lower SP value of 30.3‰ for fDNF or a lower Δδ 15 N value for the nDNF endmember, respectively; Supplementary Table 5 ) or decreased to 28% (if all nDNF derived N 2 O were to originate from NO 2 − having a positive Δ 17 O value instead of 0‰; Supplementary Table 6 ). In contrast, ammonia-oxidation contributed on average only 3–12% (via NH 2 OH decomposition) and 8–17% (via nDNF) for the base case. Consideration of cDNF (in lieu of fDNF) as the endmember having both a high SP N2O and a NO 2 − precursor required an even higher proportion of this process to satisfy mass balance ( Supplementary Table 4 ). However, two cores in this case exhibited isotopic compositions violating mass balance (those with highest SP N2O ), evidently requiring at least some contribution of fDNF (having a higher endmember SP N2O ) over cDNF. Although the LN and LOLN treatments did not involve the Δ 17 O approach, the statistically higher SP N2O values under elevated nitrate (relative to low nitrate; Fig. 3 , Supplementary Table 2 ) point to a shift in N 2 O production mechanisms in response to NO 3 − , which must have included increased contribution by fDNF and/or cDNF. Ultimately, while the precise contribution of N 2 O pathways varies depending on prescribed endmember compositions, all scenarios indicated substantial contribution by these non-traditional N 2 O production pathways. Figure 5: Relative contribution of N 2 O produced by four cycling processes as calculated by N 2 O isotope mass balance. Each bar reflects steady-state calculations using measurements from a single core incubation (two cores were incubated per site per treatment and are shown separately), considering bacterial denitrification, ammonia oxidation, nitrifier denitrification and fungal denitrification. For illustration of the relative influence that N 2 O reduction (and its associated isotope fractionation) plays in the mass balance estimates, scenarios of both low (10%, upper) and high (90%, lower) relative N 2 O consumption are considered for each core (right side axis). Contribution by processes where mass balance estimates yielded small negative values ( Supplementary Table 4 ) were considered equal to zero for this figure, with other values weighted accordingly to sum to 100%. The reader is also referred to Supplementary Table 4 for associated error in mass balance estimates calculated by Monte Carlo simulation, as well as Supplementary Tables 5 and 6 for sensitivity analyses of alternative endmember compositions. Full size image Increased N 2 O emissions from coastal systems receiving elevated NO 3 − are well documented [4] , [8] , [9] and the ‘central role’ of NO 2 − in relation to N 2 O has been emphasized by others [6] . For example, large increases in N 2 O from sediments amended with NO 2 − (relative to NO 3 − ) was previously interpreted as evidence for ‘obligate nitrite-denitrifying bacteria’ that reduce NO 2 − to N 2 O (ref. 6 ). Similarly, based on SP N2O it was concluded that N 2 O production in estuarine sediments was controlled by an as yet ‘unidentified process’ [60] having an isotopic composition consistent with more recent studies of fungal and chemodenitrification. On the basis of our results, we suggest that these previously ‘missing’ and/or ‘unidentified’ pathways likely represent non-traditional pathways including denitrification catalysed either by fungi or reactions involving Fe(II). To the degree that our sediment incubations reflect processes ongoing under natural conditions, elevated NO 3 − loading to coastal sediments appears to increase N 2 O fluxes largely through reactions involving a NO 2 − intermediate, yet also exhibiting elevated SP values. This combination of characteristics pinpoints an increased involvement of processes not regularly considered in coastal ecosystems—namely fungal and chemodenitrification. We suggest that both may represent important, yet under-appreciated sources regulating N 2 O fluxes from redox-dynamic, organic-rich environments and warrant further examination. Studies are frequently challenged by the dynamic nature of N 2 O fluxes, which are often episodic and difficult to link to specific factors or processes (for example, refs 23 , 25 ). Although our study was conducted at steady-state (enabling our assessment of fDNF and cDNF), we posit that the commonly observed patchy and dynamic nature of N 2 O fluxes may stem from a complex network of differential contribution by direct and indirect, biological and abiotic processes, including the metabolic activity of fungi and biogeochemical redox cycling of iron. In particular, compared to bacterial denitrification and/or ammonia oxidation, their especially high yields poise these processes to be important, yet under-recognized, contributors to N 2 O dynamics in many systems. Study site and experimental setup Twenty-four sediment cores were collected in August of 2013, from three intertidal sites near Königshafen on the island of Sylt in the North Sea, Germany. Sites were ∼ 100 m apart and chosen based on qualitative differences in sediment grain size and location characteristics. The ‘Schlickwatt (MD)’ and ‘Mischwatt (MX)’ sites were located inside a small lagoon, while the ‘Sandwatt (SD)’ site was more openly exposed to wind and waves ( Supplementary Fig. 1 ). Thirty intact push cores (30 cm length, 10 cm OD, 1/8″ wall thickness) were taken using polycarbonate core liners having vertical lines of silicone sealed holes (ø 3 mm) at 1-cm intervals to allow porewater collection using Rhizon samplers. Cores were retrieved leaving ∼ 10 cm of overlying water and sealed with double o-ring Delrin caps to minimize gas exchange during transport, and brought immediately back to the laboratory. In addition to the cores used for the incubations, two additional cores were used from each site for immediate microsensor profiling (O 2 , N 2 O) and pore-water extraction (‘field cores’). The remaining cores were prepared in parallel for incubations. On completion of the incubations, microsensor profiling of O 2 and N 2 O was conducted immediately followed by extraction of porewaters. Incubations The gas-tight sealed sediment cores were incubated in the dark at in situ temperatures (19 °C) in a temperature-controlled room at the Alfred Wegener Institute—Waddensee Field Station. Throughout the incubations the overlying water of the cores was continuously supplied with filtered seawater from large carboys, which were refilled as needed. The o-ring sealed core tops contained inlet/outlet fittings for continual delievery of fresh seawater through gas impermeable PEEK tubing (1/8″ OD). Peristaltic pumps were used to regulate flow rates at 1.8±0.06 ml min −1 (measured gravimetrically at each sampling point) for ∼ 8 days. The inflow line was placed near the sediment–water interface to minimized stratification. For experimental manipulations, four different inflow seawater compositions were used: ‘Low nitrate’ (air sparged; ∼ 20 μM; LN), ‘Low oxygen, low nitrate’ (sparged with N 2 to 30–35% O 2 saturation; ∼ 20 μM; LOLN), ‘High nitrate’ (amended with NaNO 3 to ∼ 120 μM (above background nitrate); HN) and ‘low oxygen, high nitrate’ (combined treatments; LOHN). Sample collection Samples of each sediment core effluent were taken twice per day. For dissolved ions, effluent was directed into HDPE bottles and allowed to fill for ∼ 60 min before subsampling, filtering (0.2 μm) and freezing (−20 °C). Separate 20 ml aliquots were taken for measurement of dissolved inorganic nitrogen concentrations (nitrate, nitrite and ammonium) and stable isotopic composition. Concentrations of nitrite and ammonium were made immediately (see below), while nitrate concentrations were measured later in the Wankel lab at WHOI. Samples for dissolved N 2 O were directed through gas impermeable PEEK tubing directly into pre-evacuated Tedlar gas sampling bags followed by gentle transfer into 160 ml serum bottles using a ¼″ OD silicone tubing, filling from the bottom to minimize turbulence and gas exchange. Sample water was allowed to overflow the bottle volume for at least two volumes before crimp-sealing with grey butyl septa and preserving with 100 μl of a saturated HgCl 2 solution. Porewater sampling Pore water samples were collected from sediment cores in 1-cm depth intervals using Rhizons [61] , which were inserted into intact sediment cores through silicon-filled ports in the walls of the core tubes. Samples of 5–10 ml volume were taken starting at the sediment–water interface down to 16 cm depth and frozen immediately for later analysis. Parallel cores were sectioned in 1-cm intervals for the analyses of iron. HCl extractable Fe(II) and the amorphous, poorly crystalline fraction of the Fe(III) minerals were measured by procedures described in ref. 63 , with the modifications as in ref. 64 . Concentration and flux measurements of N bearing species Concentrations of NO 3 − +NO 2 − were measured by chemiluminescence after reduction in a hot acidic vanadyl sulfate solution on a NOx analyser [65] . Concentrations of NO 2 − were quantified by using the Griess–Ilosvay method followed by measuring absorption 540 nm, and NO 3 − was quantified by difference [66] . Concentrations of NH 4 + were measured by fluorescence using the OPA method [62] . Concentrations of N 2 O were made using the integrated peak area of the m/z 44 beam on the IRMS (see below), standardizing to analyses of known amounts of N 2 O (injected into N 2 sparged seawater in 160 ml serum bottles) and normalizing to sample volume (158 ml). Mass fluxes ( Supplementary Fig. 2 ; Supplementary Table 1 ) were calculated as a function of the steady-state difference (usually after ∼ 3 days) between influent and effluent concentrations (Δ[ C ]), flow rate ( r ) and sediment surface area ( A ) using: Flux=(Δ[ C ] × r )/ A . Error estimates of fluxes incorporate variations in both measured flow rates as well as steady state concentrations. Isotope measurements All N and O isotopic composition measurements (δ 15 N and δ 18 O; where δ 15 N=(( 15 R sample / 15 R Air )−1) × 1,000 in units of ‰, and 15 R= 15 N/ 14 N and where δ 18 O=(( 18 R sample / 18 R VSMOW )−1) × 1,000 in units of ‰, and 18 R= 18 O/ 16 O) were made after conversion of analytes to nitrous oxide, followed by purification with a customized purge and trap system and analysis on a continuous flow IsoPrime 100 isotope ratio mass spectrometer (IRMS). Nitrate . Nitrate was converted to N 2 O using the denitrifier method [67] , [68] after removal of nitrite by addition of sulfamic acid [69] . Corrections for drift, size and fractionation of O isotopes during bacterial conversion were carried out using NO 3 − reference materials USGS 32, USGS 34 and USGS 35 (refs 67 , 70 ), with a typical reproducibility of 0.2 and 0.4‰ for δ 15 N and δ 18 O, respectively, in the course of single run. Triple oxygen isotope measurements allow for the determination of ‘anomalous 17 O,’ (the deviation from the terrestrial fractionation line) with the magnitude of this anomaly expressed as Δ 17 O (after [71] ), where: Nitrate Δ 17 O measurements were made on separate aliquots by routing denitrifier-produced N 2 O through a gold tube (1/16″ OD) held at 780 °C, thermally decomposing the N 2 O into N 2 and O 2 , which were chromatographically separated using a 2 m column (1/16″ OD) packed with molecular sieve (5 Å) before analysis on the IRMS [72] , [73] . Nitrate reference materials USGS 35 and USGS 34 were used to normalize any scale contraction during conversion, with reproducibility of Δ 17 O typically ±0.8‰. Nitrite . All samples for nitrite N and O isotope measurements were converted to N 2 O within 2 h of collection using the azide method [74] . Parallel conversions of internal nitrite standards (WILIS 10, 11 and 20) were conducted to assess potential changes in reagents with time. Internal nitrite standards were also used correct for any variations due to peak size linearity and instrumental drift, with a typical reproducibility for both δ 15 N and δ 18 O of ±0.2‰. On the basis of calibrations against isotope reference materials USGS 32, 34 and 35 for δ 15 N (ref. 75 ) and N23, N7373 and N10129 for δ 18 O (ref. 76 ), the values of WILIS 10, 11 and 20 are reported here to be −1.7, +57.1 and −7.8‰ for δ 15 N and +13.2, +8.6 and +47.6‰ for δ 18 O, respectively. Nitrite Δ 17 O measurements were made after conversion to N 2 O using the azide method and normalized using a combination of NO 2 − and NO 3 − isotopic reference materials. Δ 17 O values of NO 2 − isotope standards WILIS 10 and WILIS 11 were calibrated previously against USGS 34 and USGS 35 using the denitrifier method followed by thermal decomposition of N 2 O to N 2 and O 2 as described above—yielding Δ 17 O values of 0‰ for both. For sample NO 2 − , raw δ 17 O and δ 18 O values were first normalized for oxygen isotopic exchange with water during the azide reaction [74] using the calibrated δ 17 O and δ 18 O values of WILIS 10 and WILIS 11. During the same IRMS run, N 2 O produced from USGS 34 and USGS 35 via the denitrifier method was also thermally converted and analysed as N 2 and O 2 . Because any isotope fractionation occurring during these reactions is mass dependent (Δ 17 O is unaffected), the Δ 17 O of NO 2 − can be calculated by normalizing to Δ 17 O values of these NO 3 − standards. We disregard the small amount of oxygen isotope exchange occurring during the denitrifier method, as this would have only a small impact on the calculated Δ 17 O values. Reduced nitrogen . Total reduced nitrogen (TRN=DON+NH 4 + ) was measured in a subset of incubation cores by oxidation of the total dissolved nitrogen (TDN) pool to nitrate via persulfate digest—followed by δ 15 N analysis using the denitrifier method [77] . The δ 15 N of the TRN pool was then calculated by mass balance by subtracting the molar contribution of the measured δ 15 N of NO 3 − and NO 2 − pools to the TDN pool. On the basis of the measurement of NH 4 + concentrations, the DON flux was generally of the same magnitude as the NH 4 + flux (not shown). For use in the mass balance calculations (for estimation of the bAMO endmember Δδ 15 N value), the δ 15 N of the TRN pool was assumed to be a reasonable proxy for the δ 15 N of the NH 4 + pool. In general, this assumption had only a very small impact on the apportionment N 2 O sources by mass balance (<1%). Nitrous oxide . For dissolved N 2 O, samples were extracted from the 160 ml serum bottles using a purge and trap approach [78] . Liquid samples were quantitatively transferred from the sample bottle into a purging flask using a 20 psi He stream, followed by He-sparging ( ∼ 45 min) and cryogenic trapping using the same system described above for nitrate and nitrite derived N 2 O. Isotopic composition of the dissolved N 2 O was measured by direct comparison against the N 2 O reference tank, as no isotopic reference materials were available at the time of the analyses (USGS 51 and USGS 52 have since been publicly released: http://isotopes.usgs.gov/lab/referencematerials.html ). The composition of this tank (δ 15 N bulk =−0.7‰; δ 18 O=+39.1‰; SP N2O =−5.3‰, where SP N2O =δ 15 N(α)−δ 15 N(β) and α and β refer to the central and outer N atoms in the linear N 2 O molecule, respectively) was calibrated directly against aliquots of two previously calibrated N 2 O tanks from the Ostrom Lab at Michigan State University, having been calibrated by Tokyo Tech (Ostrom, pers. comm.). Several sample analyses of tropospheric N 2 O from the study site using this system yielded isotope values of +6.8±0.7‰ for δ 15 N bulk , +44.1±1.7‰ for δ 18 O and +17.4±2.2‰ for SP N2O (error reported as s.d. of n =6 samples). Reported values have been corrected for any size linearity effects on isotopic ratios (31/30, 45/44 and 46/44) by using a series of reference tank subsamples injected into He-purged 20 ml headspace vials using a gastight syringe. Precision for replicate analyses of this reference gas analysed as samples (that is, aliquots injected into sample vials and analysed via purge and trap) for δ 15 N is±0.3‰, for δ 18 O is ±0.4‰ and for SP N2O is ±0.8‰. The Δ 17 O of N 2 O was calculated similar to that described above for NO 2 − . After extraction and cryotrapping, the N 2 O sample is thermally decomposed to N 2 and O 2 and chromatographically separated before measurement on the IRMS. Regular analyses of N 2 O converted from NO 3 − isotope reference materials (USGS 35 and USGS 34) via the denitrifier method were made to normalize Δ 17 O values. Triple oxygen isotope tracing of N 2 O production While the δ 18 O of most terrestrial O-bearing materials tightly co-varies with δ 17 O (along the ‘terrestrial fractionation line’), atmospheric NO 3 − , stemming from reactions involving stratospheric ozone, contains a large relative excess of 17 O giving rise to a composition falling above the terrestrial fractionation line [79] (with the magnitude of this anomaly expressed as Δ 17 O; see equation 2). Since kinetic isotope effects lead to mass dependent changes in δ 17 O values approximately half as large as in δ 18 O, the Δ 17 O remains unchanged [80] , [81] , [82] . Therefore N 2 O produced from this NO 3 − (whether by bDNF, fDNF or cDNF) will retain its Δ 17 O, despite any kinetic isotope fractionation. Changes in Δ 17 O of an O-bearing N pool only occur through production incorporating O atoms having Δ 17 O ∼ 0‰ (O 2 (Δ 17 O=−0.3‰) or H 2 O (Δ 17 O=0‰) incorporated during AMO), thus, decreasing the Δ 17 O of the standing pool towards ∼ 0‰. To the degree that NO 2 − derives from NO 3 − reduction (and hence carries its Δ 17 O value), isotope equilibration between NO 2 − and water O may also ‘erase’ a non-zero Δ 17 O signal. Thus, in our incubations Δ 17 O N2O provides independent quantification of the fraction of O atoms originally deriving from NO 3 − (through a NO 2 − intermediate): Normalizing for any potential equilibration of intermediate NO 2 − with water, Δ 17 O N2O can similarly be compared to Δ 17 O of the NO 2 − pool: Isotope mass balance approach Isotope mass balance calculations were made for estimating the relative contribution of N 2 O production pathways in the sediment incubations (denitrification by bacteria (bDNF), by fungi (fDNF), or by chemodenitrification (cDNF), as well as combined production by ammonia oxidizing bacteria and archaea via NH 2 OH decomposition (AMO) or nitrifier denitrification (nDNF)). By combining four independent mass balance expressions (equations 5, 6, 9 and 11 below) we can solve for the contribution of four independent N 2 O production processes (here we describe consideration of fDNF (case 1), with cDNF being considered separately (case 2)). Equation 1 can be expressed in terms of the fractional contribution (f) of each production process to the total flux of N 2 O: Equation 4, incorporating the Δ 17 O measurements, is used but neglecting cDNF for this case: For measured Δδ 15 N values, equation 7 describes the mass balance contribution of each process to the cumulative steady-state flux (Δδ 15 N meas ): where again f refers to the fractional contribution of a given process, Δδ 15 N is equal to the steady-state difference (or offset) between δ 15 N of NO 3 − and N 2 O, and where the endmember Δδ 15 N for given process is expressed based on measured steady-state δ 15 N values of NO 3 − , NO 2 − or NH 4 + and the isotope offsets for each process ( Supplementary Table 3 ). For example, the difference between δ 15 N of reactant NH 3 and N 2 O ( 15 ɛ NH3-N2O ) produced by bAMO has been estimated to be ∼ 3.7±3‰, with δ 15 N N2Obulk depleted in 15 N relative to the NH 3 source [59] . To express this in terms of a Δδ 15 N value for the NO 3 − /N 2 O mass balance in equation 7, we also need to account for the steady-state difference between the δ 15 N of NO 3 − and NH 4 + such that: As the isotopic composition of N 2 O from bAMO and aAMO are very similar in the context of the isotope space evaluated here [56] , [57] , [58] , we choose to combine these terms into a single term (AMO), having the composition of bAMO ( Supplementary Table 3 ). Together with the fact that we will treat cDNF separately, equation 7 thus simplifies to: Similar to equation 7, the fractional contribution of each process to the measured SP N2O of the effluent can be expressed as: where f denotes the fractional contribution of a given process having a particular SP value, and where f(N 2 O RED ) is equal to 1−(F N2O /(F bDNF +F fDNF +F cDNF +F bAMO +F aAMO +F nDNF )) and SP ɛ N2ORED is the kinetic isotope effect on SP for N 2 O reduction of −6‰ (refs 21 , 22 ). As in equation 9, consideration of four processes simplifies equation 10 to: By combining equations 5, 6, 9 and 11—we can uniquely solve for the fractional contribution of four processes (bDNF, fDNF, AMO and nDNF) to the total observed N 2 O fluxes of the core incubations ( Fig. 5 ; Supplementary Table 4 ). Isotope offsets (Δδ 15 N) and SP N2O values for defining endmember compositions are given in Supplementary Table 3 , as well as the expected Δ 17 O N2O /Δ 17 O NO2 values for the high nitrate incubations. Error propagation and sensitivity analysis Error estimates for these mass balance calculations ( Supplementary Tables 4,5 and 6 ) were calculated using a Monte Carlo error propagation approach in R (with 10,000 simulations), in which randomized Gaussian distributions of values were generated, as defined by their mean and s.d. given in Supplementary Table 3 . This approach takes into account both the error associated with measurement of steady-state isotopic compositions ( Supplementary Table 2 ; which implicitly incorporates both analytical error during instrument measurement, as well as natural variability during operation of the incubations) as well as error associated with the definition of endmembers ( Supplementary Table 3 ). Beyond these estimates of error, we also evaluated the sensitivity of specific endmember values to the calculated mass balance estimates—focusing on variations for endmember values having the least amount of certainty. First, the endmember values of Δδ 15 N for bDNF and fDNF (and cDNF) are prescribed to be low as an inferred consequence of diffusion-limited expression of intrinsic (enzyme level) isotope effects ( Supplementary Table 3 ). For nDNF, we chose to use a Δδ 15 N value established by a study of nitrifiers under varying oxygen tension (Frame and Casciotti [59] ), as nitrifiers will be growing at the sharp oxic/anoxic interface in our sediment core incubations. Whether their supply of NO 2 − (as a substrate for nDNF) could be considered to be limited by diffusion is perhaps a matter of debate. However, we reasoned that nitrifiers will most generally be denitrifying the product NO 2 − that they themselves are producing (for detoxification) and therefore would not be limited by diffusion of NO 2 − from anoxic depths below. Further, the positive flux of NO 2 − out of the sediments—also indicates that the diffusive supply of NO 2 − should not have been limited (regardless of the source of the NO 2 − ). Nevertheless, we discretely examined the impact that these assumptions make by decreasing the endmember Δδ 15 N value for nDNF from 56.9 to 28‰ and then to 14‰. Under these scenarios (assuming 10% N 2 O reduction, for example)—the average relative contribution of nDNF increases from 8 to 14 and 26%, respectively, though mostly at the expense of bDNF, which decreases on average from 45 to 38 and 25%, respectively. In comparison, these scenarios actually increase estimated contribution of fDNF from 36 to 43 and 56%, respectively ( Supplementary Table 5 ). Endmember SP values have been generally well established for bDNF, nDNF and bAMO through culture studies under a variety of growth conditions. SP for fungal DNF is admittedly less well studied, however, several studies have shown that SP values are universally elevated (often clustering ∼ 35–37‰). Recent studies [37] , [42] observe that most N 2 O producing fungal cultures yielded SP values >30‰. Finally, even the purified N 2 O producing fungal enzyme (p450nor) has been shown to exhibit elevated SP values, albeit at somewhat lower values (15–29‰). Notably, our choice of +37‰ for the fDNF endmember is conservative in estimation of the relative contribution of fDNF. For example, decreasing this value to the mean reported by Maeda et al . [37] of +30.3±4.8‰ (which notably also contained some questionably low values), results in an average of a 6% increase in the contribution of fDNF to N 2 O production, with the average contribution of 36% shifting up to an average of 41–42% ( Supplementary Table 6 ). Finally, we evaluated our assumption that the extracellular NO 2 − pool could be disregarded as a reactant source for nDNF (that in situ , nDNF only occurred from NO 2 − supplied via bAMO), by setting the prescribed Δ 17 O-N 2 O/Δ 17 O-NO 2 − value for nDNF to a value of ‘1’ instead of ‘0’—representing the most extreme case. Indeed, under this scenario—the average estimated contribution of bNDF and nDNF actually do not change by > ∼ 1%, while bAMO is increased (from 12 to 19%) and fDNF is decreased (from 36 to 28%) ( Supplementary Table 6 ). Fungal genetic sequencing Sediment samples for fungal sequence analysis were collected and stored frozen at −80 °C. Genomic DNA from marine sediment samples was extracted using a bead beating protocol according to the manufacturer’s instruction (Mo Bio, Carlsbad, CA). ITS region sequences were amplified using the fungal ITS primer pair F (ITS5): GGAAGTAAAAGTCGTAACAAGG and R (ITS4): TCCTCCGCTTATTGATATGC generating fragments of ∼ 600 bps in length. PCR products were cloned using Zero Blunt TOPO PCR Cloning (Thermo Fisher, Carlsbad, CA). After a ligate buffer exchange the plasmid was transferred into TOP10 electrocompetent cells. Cells were plated and grown on LB agar containing kanamycin. Single colonies were recovered from each plate and amplified using M13F&R primers. The products were sequenced by Sanger method (EtonBio, San Diego, CA). Sequences were analysed using BLAST. Taxonomy was assigned for fungal sequences ( Supplementary Figure S3 ) by comparison against untrimmed ITS in the UNITE database (01/08/2015 version), using QIIME v1.91. Sequences were assigned only if the database match had a similarity of at least 90% and maximum e-value of 0.001. Data availability The data sets generated during this study are available by request from corresponding author. How to cite this article: Wankel, S. D. et al . Evidence for fungal and chemodenitrification based N 2 O flux from nitrogen impacted coastal sediments. Nat. Commun. 8 , 15595 doi: 10.1038/ncomms15595 (2017). Publisher’s note: Springer Nature remains neutral with regard to jurisdictional claims in published maps and institutional affiliations.